Regulatory network decoded from epigenomes of surface ectoderm-derived cell types Developmental history shapes the epigenome and biological function of differentiated cells. Epigenomic patterns have been broadly attributed to the three embryonic germ layers. Here we investigate how developmental origin influences epigenomes. We compare key epigenomes of cell types derived from surface ectoderm (SE), including keratinocytes and breast luminal and myoepithelial cells, against neural crest-derived melanocytes and mesoderm-derived dermal fibroblasts, to identify SE differentially methylated regions (SE-DMRs). DNA methylomes of neonatal keratinocytes share many more DMRs with adult breast luminal and myoepithelial cells than with melanocytes and fibroblasts from the same neonatal skin. This suggests that SE origin contributes to DNA methylation patterning, while shared skin tissue environment has limited effect on epidermal keratinocytes. Hypomethylated SE-DMRs are in proximity to genes with SE relevant functions. They are also enriched for enhancer- and promoter-associated histone modifications in SE-derived cells, and for binding motifs of transcription factors important in keratinocyte and mammary gland biology. Thus, epigenomic analysis of cell types with common developmental origin reveals an epigenetic signature that underlies a shared gene regulatory network. Although epigenetic mechanisms are crucial in establishing and maintaining cell identity, the role of developmental origin and tissue microenvironment in shaping the epigenome is just beginning to be unraveled. Marked epigenomic transitions occur on directed embryonic stem cell (ESC) differentiation into the three major embryonic lineages [1] , [2] and over the course of development [3] . Differentiated cells and tissues have specific DNA hypomethylation signatures, particularly at enhancers [4] , [5] ; however, a subset of hypomethylated enhancers are actually dormant in adult tissues and are active only in corresponding fetal tissues, suggesting that a DNA methylation memory of fetal origin may be retained in adult cells [6] . Similarly, DNase I-hypersensitive patterns in differentiated cells can reflect embryonic lineage and mark a subset of embryonic enhancers [7] . Tissue microenvironment influences cell identity and morphogenesis [8] , and consequently may affect epigenomes. Accordingly, perturbation of tissue microenvironment is associated with epigenomic alteration [9] , [10] . These studies suggest that embryonic origin and tissue environment may influence normal cellular epigenomic states and that differentiated cell epigenomes can be used to infer epigenomic patterns of precursor embryonic cell populations. To investigate how developmental origin and tissue environment contribute to cell type-specific epigenetic patterns, we use the skin as a model system. The three most prevalent skin cell types are each derived from a different embryonic origin (keratinocytes from surface ectoderm (SE), fibroblasts from mesoderm and melanocytes from neural crest [11] ), but exist within a shared tissue environment ( Fig. 1 ). We generate DNA methylation and histone modification profiles for these three skin cell types and compare their epigenomes among the skin cell types and against breast, blood and brain tissue epigenomes. The three skin cell types share few regions with common DNA- methylation and histone modification states, which are not present in the other tissue samples. SE-derived skin keratinocytes and breast cells, however, share many common differentially DNA methylated regions (SE-DMRs). SE-DMRs enrich for enhancer- and promoter-associated histone modifications in SE-derived cell types and for binding motifs of relevant transcription factors. Reconstruction of the gene regulatory network connecting these transcription factors and putative target genes with nearby SE-DMRs demarcate epigenetic and regulatory events associated with structural components and signalling pathways in SE-derived cell types. Thus, for SE-derived cells, their shared developmental origin influences their epigenomes to a greater extent than tissue environment. Furthermore, a shared gene regulatory network emerge from the SE-DMR signature. 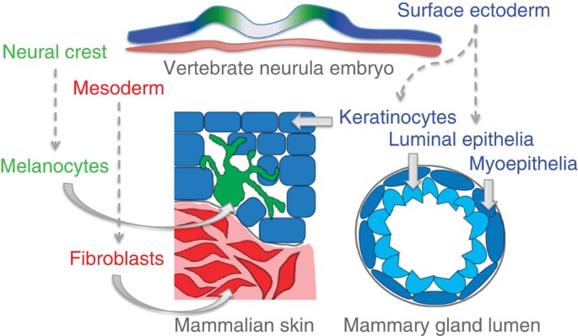Figure 1: Developmental origins of samples. Developmental origins of skin and breast cell types used in this study. Embryonic surface ectoderm from the vertebrate neurula stage embryo (blue) gives rise to keratinocytes in the skin and cells of the mammary gland lumen. Embryonic neural crest cells (green) will produce melanocytes that intercalate with epidermal keratinocytes. Skin fibroblasts are derived from embryonic mesoderm (red). Figure 1: Developmental origins of samples. Developmental origins of skin and breast cell types used in this study. Embryonic surface ectoderm from the vertebrate neurula stage embryo (blue) gives rise to keratinocytes in the skin and cells of the mammary gland lumen. Embryonic neural crest cells (green) will produce melanocytes that intercalate with epidermal keratinocytes. Skin fibroblasts are derived from embryonic mesoderm (red). Full size image Skin cell type-specific differentially methylated regions Fibroblasts, melanocytes and keratinocytes were individually isolated from each of three neonatal human foreskins and expanded as short-term primary cultures. From these samples, we generated nine high-resolution epigenomes encompassing key histone modifications (H3K4me1, H3K4me3 and H3K27ac) and DNA methylation, along with messenger RNA and microRNA (miRNA) expression profiles ( Supplementary Data 1 and 2 ). The effects of ageing and environmental exposure were minimized by using neonatal samples. As each set of three cell types shares a common genome, the effect of genetic variation on epigenetic variability was also minimized. We identified 12,892 regions encompassing 193,202 CpGs with a DNA methylation status unique to one of the three skin cell types and consistent across all three individuals (Methods, Fig. 2a , Supplementary Figs 1–3 and 4a , Supplementary Notes 1–3 and Supplementary Table 1 ). The majority of these skin cell type-specific DMRs were hypomethylated ( Fig. 2a ), suggesting potential cell type-specific regulatory activity at these regions [4] , [12] , [13] . Forty to 46% of the DMRs were intergenic and 5–9% were associated with RefSeq-annotated gene promoters ( Supplementary Fig. 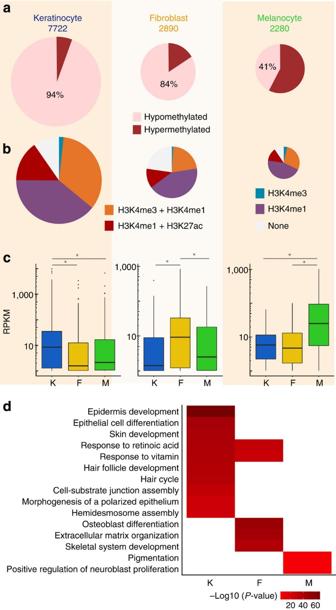Figure 2: Identification and characterization of skin cell type-specific DMRs. (a) Hypomethylation and hypermethylation percentages for each set of skin cell type-specific DMRs defined by comparison against the other two skin cell types. The total number for each set of cell type-specific DMRs is listed above the pie chart. DMRs are 500 bp windows. (b) Histone modification patterns at skin cell type-specific hypomethylated DMRs. (c) Skin cell-type RNA expression levels for genes with hypomethylated cell type-specific DMRs in their promoter regions. Each panel depicts expression values for a set of cell type-specific DMR-associated genes. Plotted values are RNA-seq RPKM values over exons, averaged (mean) over three biological replicates. For each box plot, the middle line indicates the median value, top and bottom box edges are the third- and first-quartile boundaries, respectively. The upper whisker is the highest data value within 1.5 times the interquartile range; the lower whisker indicates the lowest value within 1.5 times the interquartile range. The interquartile range is the distance between the first and third quartiles. Points indicate data beyond whiskers. Logarithmic scale transformations were applied before box plot statistics were computed. RPKM distributions for a given set of cell type-specific DMR-associated genes in the specified cell type compared with other cell types were statistically significant (Wilcoxon ranked test, paired, *P-value≪0.003, Keratinocyte-DMRsn=602, Fibroblast-DMRsn=108, Melanocyte-DMRsn=74; K, keratinocytes; F, fibroblasts; M, melanocytes;Supplementary Tables 3–5). (d) Heat map depicting selected GO terms enriched for keratinocyte, fibroblast and melanocyte-hypomethylated cell type-specific DMRs. F, fibroblasts; K, keratinocytes; M, melanocytes. Colour intensity represents the negative log10 transformedP-value of enrichment of a given cell type-specific DMR set for association with the listed GO term. Full data sets are inSupplementary Data 3. 5 ); non-CpG island promoters were enriched among cell type-specific DMRs ( Supplementary Note 4 and Supplementary Table 2 ). Eighty to 91% of hypomethylated cell type-specific DMRs overlapped with regulatory element-associated histone modifications in the same cell type ( Fig. 2b ). Accordingly, hypomethylation of cell type-specific DMRs at gene promoters correlated with increased gene expression relative to the other two cell types where the DMR was hypermethylated ( Fig. 2c and Supplementary Tables 3–5 ). Gene Ontology (GO) analysis using the GREAT (ref. 14 ) tool on hypomethylated cell type-specific DMRs showed strong enrichment for biological processes relevant to each cell type (for example, ‘extracellular matrix organization’ for fibroblasts ( P -value=9.05E−45) and ‘pigmentation’ for melanocytes ( P -value=2.43E−06); Fig. 2d and Supplementary Data 3 ). These data suggest skin cell type-specific DMRs occur primarily at distal enhancers and regulate genes relevant to each cell type. Figure 2: Identification and characterization of skin cell type-specific DMRs. ( a ) Hypomethylation and hypermethylation percentages for each set of skin cell type-specific DMRs defined by comparison against the other two skin cell types. The total number for each set of cell type-specific DMRs is listed above the pie chart. DMRs are 500 bp windows. ( b ) Histone modification patterns at skin cell type-specific hypomethylated DMRs. ( c ) Skin cell-type RNA expression levels for genes with hypomethylated cell type-specific DMRs in their promoter regions. Each panel depicts expression values for a set of cell type-specific DMR-associated genes. Plotted values are RNA-seq RPKM values over exons, averaged (mean) over three biological replicates. For each box plot, the middle line indicates the median value, top and bottom box edges are the third- and first-quartile boundaries, respectively. The upper whisker is the highest data value within 1.5 times the interquartile range; the lower whisker indicates the lowest value within 1.5 times the interquartile range. The interquartile range is the distance between the first and third quartiles. Points indicate data beyond whiskers. Logarithmic scale transformations were applied before box plot statistics were computed. RPKM distributions for a given set of cell type-specific DMR-associated genes in the specified cell type compared with other cell types were statistically significant (Wilcoxon ranked test, paired, * P- value ≪ 0.003, Keratinocyte-DMRs n =602, Fibroblast-DMRs n =108, Melanocyte-DMRs n =74; K, keratinocytes; F, fibroblasts; M, melanocytes; Supplementary Tables 3–5 ). ( d ) Heat map depicting selected GO terms enriched for keratinocyte, fibroblast and melanocyte-hypomethylated cell type-specific DMRs. F, fibroblasts; K, keratinocytes; M, melanocytes. Colour intensity represents the negative log10 transformed P -value of enrichment of a given cell type-specific DMR set for association with the listed GO term. Full data sets are in Supplementary Data 3 . Full size image Skin tissue-specific epigenomic features We next examined whether the common tissue environment of the three skin cell types would impose an identifiable skin tissue epigenetic signature. For comparison, we generated complete epigenomes and transcriptomes for a panel of non-skin cell types and tissues (including brain tissue and breast and blood cell types) and identified DMRs shared by all three skin cell types relative to other tissues ( Supplementary Fig. 4b and Supplementary Note 5 ). Of the 28,776 total DMRs detected, only 8 regions shared the same methylation status in skin cell types and the opposite methylation status in all other samples ( Fig. 3a,b ). Hierarchical clustering based on methylation levels at the 28,776 DMRs reveals that although samples of the same cell type cluster together, the three skin cell types do not ( Fig. 3c ). These results suggested that skin cell-type methylomes did not share many differences compared with breast, brain and blood cell methylomes, and that skin tissue lacks a specific and substantive DNA methylation signature. 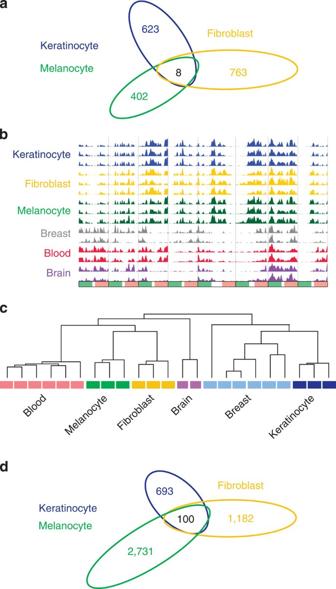Figure 3: Skin-tissue level epigenomic features. (a) Venn diagram showing number of DMRs for each of the skin cell types compared with non-skin samples (brain, breast and blood). Eight DMRs (overlap region) share the same methylation status in the three skin cell types and have the opposite methylation status in all non-skin samples. (b) WashU Epigenome Browser screenshot of the eight DMRs where the three skin cell types share the same methylation status and all non-skin cell types have the opposite methylation status. Each column represents a 500-bp window ±2.5 kb, except for two columns that represent multiple contiguous 500 bp windows ±2.5 kb. Each row is a MeDIP-seq track for the indicated cell type. Three replicates for each skin cell type and two replicates for each non-skin sample are depicted. (c) Clustering dendrogram based on average DNA methylation levels (predicted by methylCRF44) at 28,776 DMRs found between skin and brain tissue, breast and blood cell types. (d) Venn diagram showing number of H3K4me1 peaks for each skin cell type that are absent in all non-skin samples (brain, breast and blood), which also have overlapping H3K27ac signal. The intersection represents the 100 overlapping regions where H3K4me1 and H3K27ac peaks are present in all three skin cell types and H3K4me1 peaks are absent in all non-skin samples. Figure 3: Skin-tissue level epigenomic features. ( a ) Venn diagram showing number of DMRs for each of the skin cell types compared with non-skin samples (brain, breast and blood). Eight DMRs (overlap region) share the same methylation status in the three skin cell types and have the opposite methylation status in all non-skin samples. ( b ) WashU Epigenome Browser screenshot of the eight DMRs where the three skin cell types share the same methylation status and all non-skin cell types have the opposite methylation status. Each column represents a 500-bp window ±2.5 kb, except for two columns that represent multiple contiguous 500 bp windows ±2.5 kb. Each row is a MeDIP-seq track for the indicated cell type. Three replicates for each skin cell type and two replicates for each non-skin sample are depicted. ( c ) Clustering dendrogram based on average DNA methylation levels (predicted by methylCRF [44] ) at 28,776 DMRs found between skin and brain tissue, breast and blood cell types. ( d ) Venn diagram showing number of H3K4me1 peaks for each skin cell type that are absent in all non-skin samples (brain, breast and blood), which also have overlapping H3K27ac signal. The intersection represents the 100 overlapping regions where H3K4me1 and H3K27ac peaks are present in all three skin cell types and H3K4me1 peaks are absent in all non-skin samples. Full size image To determine whether skin tissue also lacks a shared histone modification signature, we identified cell type-specific chromatin states from H3K4me1, H3K4me3 and H3k27ac chromatin immunoprecipitation sequencing (ChIP-seq) data for each skin cell type, as well as for breast, brain and blood samples. Among the 259,297 enhancer-associated H3K4me1 peaks and 55,859 promoter-associated H3K4me3 peaks identified in the above samples, only 997 H3K4me1 and 57 H3K4me3 peaks are present in all three skin cell types and absent in the other samples ( Supplementary Figs 6 and 7 ). Only 100 of the 997 exclusively skin-specific H3K4me1 peaks overlapped with H3K27ac peaks (a combination which marks active enhancers) in all three skin cell types ( Fig. 3d ). Although GO enrichment analysis for cell type-specific histone modification patterns showed enrichment for relevant terms, analysis for the few exclusively skin tissue-shared histone modification peaks did not reveal any relevant enrichment ( Supplementary Data 4 ). The minimal DNA methylation and histone modification commonalities that separate skin cell types from other tissues and the lack of functional enrichment for these common shared regions strongly suggest that the shared skin tissue environment does not significantly influence its constituent cell-type epigenomes at this developmental stage. Developmental origin influences epigenomes In the absence of a strong skin tissue-specific epigenetic signature, we hypothesized that developmental origin is a major determinant of skin cell-type epigenetic patterns. We explored this hypothesis by focusing on skin keratinocytes and breast epithelial cells, which are both derived from SE [15] . Consistent with their shared developmental origin, neonatal skin keratinocytes clustered with adult breast epithelial cell types based on DNA methylation values at the DMRs previously identified in skin and non-skin cell pairwise comparisons ( Fig. 3c ). To specifically define the DNA methylation signature of SE-derived cell types, we identified DMRs for each of the surface ectodermal cell types in a pairwise manner compared with neonatal skin melanocytes and fibroblasts, which are derived from other embryonic germ layers ( Supplementary Fig. 4c ). There were 1,392 DMRs with the same methylation state exclusively in keratinocyte, breast myoepithelial and breast luminal epithelial cells relative to the two other cell types, which we inferred to be SE-specific DMRs (SE-DMRs) (Methods and Fig. 4a ). Therefore, common developmental origin influences SE-derived cell epigenomes to a greater extent than does the shared skin tissue environment. 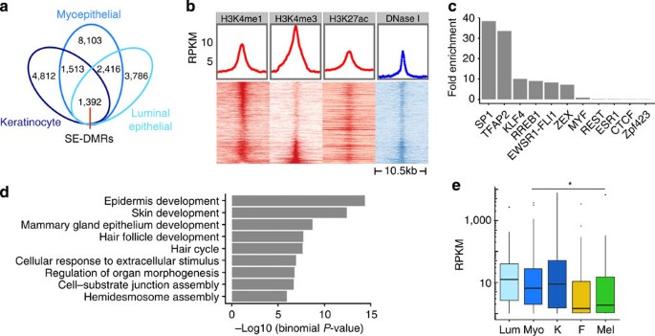Figure 4: Identification and characterization of SE-DMRs. (a) Venn diagram showing SE-specific DMRs, defined as the overlap of keratinocyte, breast myoepithelial and luminal epithelial cell DMRs. (b) Enrichment of H3K4me1, H3K4me3, H3K27ac and DNAse I-hypersensitivity at SE-DMRs in one keratinocyte sample replicate. Each heat map column represents histone modification ChIP-seq or DNAse-seq signal at 500 bp SE-DMRs ±5 kb. Each heat map row represents a single hypomethylated SE-DMR, ordered by decreasing H3K4me1 signal, then increasing H3K4me3 signal. (c) Bar plot of enrichment values for top ten enriched TFBS motifs determined by motif scanning of hypomethylated SE-DMRs using FIMO47(Methods). Enrichment based on hg19 genome background. (d) Selected GO terms enriched for hypomethylated SE-DMRs.P-value of enrichment calculated by GREAT14. Full list of enriched GO terms is inSupplementary Data 5. (e) Box plots showing RNA expression levels for genes with hypomethylated SE-DMRs in promoter regions. Skin cell-type RNA-seq RPKM values over exons are averages (mean) of three biological replicates; luminal epithelial and myoepithelial values are a single biological replicate. The middle line indicates the median value, top and bottom box edges are the third- and first-quartile boundaries, respectively. The upper whisker is the highest data value within 1.5 times the interquartile range; the lower whisker indicates the lowest value within 1.5 times the interquartile range. The interquartile range is the distance between the first and third quartiles. Points indicate data beyond whiskers. Logarithmic scale transformation was applied before box plot statistics were computed. RPKM distributions for SE cell-type expression levels versus non-SE cell-type expression levels are statistically significant (Wilcoxon-ranked test, paired, *P-value≪0.02;n=150 genes) (F, fibroblasts; K, keratinocytes; Lum, breast luminal epithelial cells M, melanocytes; Myo, breast myoepithelial cells;Supplementary Table 6). Figure 4: Identification and characterization of SE-DMRs. ( a ) Venn diagram showing SE-specific DMRs, defined as the overlap of keratinocyte, breast myoepithelial and luminal epithelial cell DMRs. ( b ) Enrichment of H3K4me1, H3K4me3, H3K27ac and DNAse I-hypersensitivity at SE-DMRs in one keratinocyte sample replicate. Each heat map column represents histone modification ChIP-seq or DNAse-seq signal at 500 bp SE-DMRs ±5 kb. Each heat map row represents a single hypomethylated SE-DMR, ordered by decreasing H3K4me1 signal, then increasing H3K4me3 signal. ( c ) Bar plot of enrichment values for top ten enriched TFBS motifs determined by motif scanning of hypomethylated SE-DMRs using FIMO [47] (Methods). Enrichment based on hg19 genome background. ( d ) Selected GO terms enriched for hypomethylated SE-DMRs. P -value of enrichment calculated by GREAT [14] . Full list of enriched GO terms is in Supplementary Data 5 . ( e ) Box plots showing RNA expression levels for genes with hypomethylated SE-DMRs in promoter regions. Skin cell-type RNA-seq RPKM values over exons are averages (mean) of three biological replicates; luminal epithelial and myoepithelial values are a single biological replicate. The middle line indicates the median value, top and bottom box edges are the third- and first-quartile boundaries, respectively. The upper whisker is the highest data value within 1.5 times the interquartile range; the lower whisker indicates the lowest value within 1.5 times the interquartile range. The interquartile range is the distance between the first and third quartiles. Points indicate data beyond whiskers. Logarithmic scale transformation was applied before box plot statistics were computed. RPKM distributions for SE cell-type expression levels versus non-SE cell-type expression levels are statistically significant (Wilcoxon-ranked test, paired, * P -value ≪ 0.02; n =150 genes) (F, fibroblasts; K, keratinocytes; Lum, breast luminal epithelial cells M, melanocytes; Myo, breast myoepithelial cells; Supplementary Table 6 ). 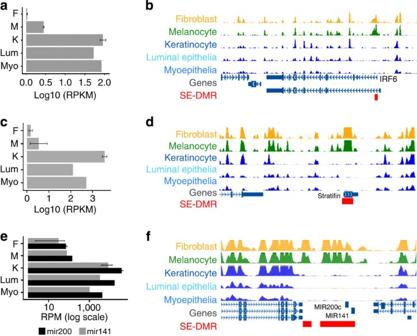Figure 6: RNA expression levels and browser screenshots of selected loci with SE-DMRs. (a) Expression values forIRF6in each cell type as listed on the left;xaxis is expression values in log10-transformed RPKM for each cell type. Skin cell-type values are averages (mean) of three biological replicates (error bars are s.e.m.); luminal epithelial and myoepithelial values are a single biological replicate. (b) Browser screenshot ofIRF6locus and surrounding genomic region. MeDIP-seq tracks are shown for the indicated cell types; all trackyaxes heights are 60 RPKM. Red box, hypomethylated SE-DMR near theIRF6promoter. (c) Expression for Stratifin (SFN) as ina. (d) Browser screenshot ofSFNlocus. Tracks as inb. Red box, hypomethylated SE-DMR atSFNpromoter. (e) Expression values for mir-200c and mir-141 in each cell type as listed to the left;xaxis is reads per million (RPM, log scale). Keratinocyte value is the average (mean) of three biological replicates; fibroblast value is the mean of two biological replicates, (error bars are s.e.m.); melanocyte, luminal epithelial and myoepithelial values are a single biological replicate. (f) Browser screenshot of mir-200c/mir-141 locus and surrounding genomic region. Tracks as inb. Red boxes, hypomethylated SE-DMRs including and adjacent to both miRNA loci. Full size image We examined whether SE-DMRs, similar to cell-type-specific DMRs, possessed regulatory potential. The majority (97%) of SE-DMRs were hypomethylated with 12% located in gene promoters and 40% within intergenic regions ( Supplementary Fig. 8a ). Hypomethylated SE-DMRs were enriched for promoter- and enhancer-associated histone modifications in both keratinocytes and breast myoepithelial cells, and for DNase I-hypersensitive sites in keratinocytes ( Fig. 4b and Supplementary Fig. 8b ). Hypomethylated SE-DMRs were also enriched for transcription factor binding motifs including TFAP2 and KLF4 ( Fig. 4c ); transcription factors that bind to these two motifs function in keratinocyte and mammary epithelium development, differentiation and/or maintenance of cell fate [16] , [17] , [18] , [19] , [20] . Genes associated with hypomethylated SE-DMRs were enriched for functions relevant to the biology of these cell types, such as ‘epidermis development’ ( P -value=4.35e−15) and ‘mammary gland epithelium development’ ( P -value=2.10e−9) ( Fig. 4d and Supplementary Data 5 ). DNA hypomethylation status of genes with hypomethylated SE-DMRs in their promoter regions correlated with increased expression in SE-derived cells relative to non-SE cells ( Fig. 4e and Supplementary Table 6 ). These annotations suggested that the majority of SE-DMRs were at distal enhancer or gene promoter elements and regulate genes important for keratinocyte and mammary gland development. More generally, these results offer a new and deeper level of interrogating the origin and function of adult epigenomes, adding significantly to the recent attribution of epigenome signatures to germinal layers [1] , [2] . Epigenome-derived SE regulatory network Given their regulatory element signatures, overlap with DNase I-hypersensitive sites and enrichment for relevant transcription factor binding site (TFBS) motifs, we hypothesized that hypomethylated SE-DMRs may be regulatory elements that coordinate expression of genes essential for function of SE-derived cells. To test this, we sought to connect these putative regulatory elements to genes in a SE gene network. We associated DMRs with nearby putative target genes and queried databases of TF-target genes and gene–gene interactions to construct regulatory relationships among these genes (Methods). The result is a highly connected network with a statistically significant number of connections (1458 edges, 278 nodes; P- value=1.25e−4; Methods, Supplementary Data 6 and Supplementary Table 7 ), whose distribution follows a power law ( R 2 =0.89; Supplementary Fig. 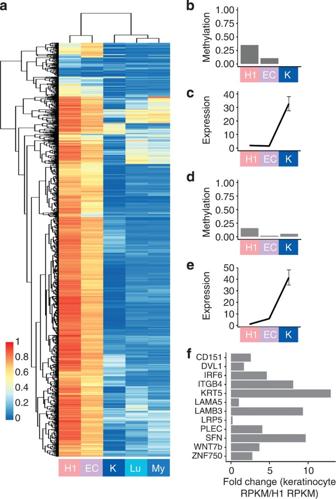Figure 7: DNA methylation dynamics of SE-DMRs across samples from different developmental stages. (a) Heatmap and clustering dendrogram based on average CpG DNA methylation values of hypomethylated SE-DMRs for different developmental samples. Each row represents one of 1,307 DMRs for which there are CpGs with ≥10 × coverage in WGBS data. Methylation values for H1 ESCs, ectoderm differentiated ESCs (‘EC’) and keratinocyte (‘K’) are from WGBS; breast luminal (‘Lu’) and myoepithelial (‘My’) values are the average of single CpG methylCRF predictions in each DMR. MethylCRF predictions are based on MeDIP-seq and MRE-seq data for these samples (Methods). A value of ‘1’ is fully methylated; ‘0’ is completely unmethylated. (b)KLF4gene body SE-DMR average CpG DNA methylation levels across developmental stages. (c)KLF4RNA expression across developmental stages. Values are RPKM over coding exons; error bars for keratinocytes are s.e.m.,n=3. Sample abbreviations as ina. (d)TFAP2Apromoter SE-DMR average CpG DNA methylation levels across developmental stages. (e)TFAP2ARNA expression across developmental stages. Values are RPKM over coding exons; error bars for keratinocytes are s.e.m.,n=3. Sample abbreviations as ina. (f) RNA expression levels in keratinocytes relative to H1 ESCs for selected genes with hypomethylated SE-DMRs in their promoters. These SE-DMRs, as in the majority of hypomethylated SE-DMRs, were methylated in H1 and ectoderm-differentiated ESCs but lowly methylated in differentiated SE cell types. Increased expression relative to an earlier developmental sample suggests these DMRs are transcriptional regulatory regions for their associated genes. 9 ). Strikingly, the transcription factors near the top of the inferred SE network were those whose motifs were enriched in the hypomethylated SE-DMRs ( Fig. 4c ). This observation, along with the network connectivity data, suggested that TFAP2a, TFAP2c and KLF4 may regulate many of the downstream genes in this network. To identify biological processes associated with each set of hypomethylated DMRs containing either TFAP2 or KLF4 TFBSs, we performed GREAT analysis [14] . The network was characterized by two partially overlapping major branches (summarized data in Fig. 5a and Supplementary Table 8 ). The first branch included the transcription factors TFAP2a and TFAP2c, and connected to genes associated with SE-relevant GO terms, for example, ‘hemidesmosome assembly’, which is a structural complex critical for epithelial cells [21] , and Notch signalling, which functions in mammary cell fate commitment [22] and keratinocyte homeostasis [23] ( Fig. 5b ). The second branch was characterized by KLF4 and was associated with mammary gland development and Wnt signalling, which influences both breast and keratinocyte cell fate decisions [24] , [25] ( Fig. 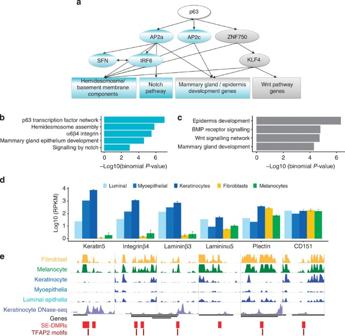5c ). Thus, we observed a highly structured set of connections between regulatory elements and putative target genes that underlie and integrate signalling pathways vital for both keratinocyte and mammary gland epithelial cell function. Figure 5: SE-DMRs are regulatory elements in a gene network. (a) Summary of the TF-target gene regulatory network derived from SE-DMR analyses. The categories at the bottom of the panel represent enriched biological processes or pathways for genes associated with DMRs containingTFAP2 or KLF4 motifs. TFAP2-associated TFs/pathways highlighted in blue; KLF4-associated pathways in grey. (b) Functional enrichment for TFAP2 motif containing hypomethylated SE-DMRs. (c) Functional enrichment for KLF4 motif containing hypomethylated SE-DMRs. (d) RNA expression values for SE-DMR associated hemidesmosome/basement membrane genes for SE and non-SE cell types. Skin cell-type values are averages (mean) of three biological replicates. Error bars are s.e.m. (e) WashU Epigenome Browser screenshot of hemidesmosome/basement membrane genes. MeDIP-seq tracks depicted in green, yellow and blue; all trackyaxes heights are 60 RPKM. DNase-seq track is shown in light blue. Genes depicted as black lines. SE-DMRs depicted as red boxes and TFAP2 motifs as maroon lines. Figure 5: SE-DMRs are regulatory elements in a gene network. ( a ) Summary of the TF-target gene regulatory network derived from SE-DMR analyses. The categories at the bottom of the panel represent enriched biological processes or pathways for genes associated with DMRs containingTFAP2 or KLF4 motifs. TFAP2-associated TFs/pathways highlighted in blue; KLF4-associated pathways in grey. ( b ) Functional enrichment for TFAP2 motif containing hypomethylated SE-DMRs. ( c ) Functional enrichment for KLF4 motif containing hypomethylated SE-DMRs. ( d ) RNA expression values for SE-DMR associated hemidesmosome/basement membrane genes for SE and non-SE cell types. Skin cell-type values are averages (mean) of three biological replicates. Error bars are s.e.m. ( e ) WashU Epigenome Browser screenshot of hemidesmosome/basement membrane genes. MeDIP-seq tracks depicted in green, yellow and blue; all track y axes heights are 60 RPKM. DNase-seq track is shown in light blue. Genes depicted as black lines. SE-DMRs depicted as red boxes and TFAP2 motifs as maroon lines. Full size image Surface ectoderm hypomethylated DMRs were located near the transcription start sites (TSSs) of six genes that encode hemidesmosome/epidermal basement membrane zone components, five of which contain the TFAP2 TFBS motif ( Fig. 5e ). These genes were highly expressed in all surface ectodermal cell types ( Fig. 5d ). Mutations occur in any one of five of these genes in various forms of the inherited epidermolysis bullosa blistering skin diseases [26] , [27] . These findings suggest SE-DMRs may coordinately regulate a suite of genes that encode for components of a key structural complex in SE-derived cells, which when perturbed leads to a clinically relevant phenotype. Hypomethylated SE-DMRs containing TFAP2 motifs were also identified near the transcription start site of two genes, IRF6 and Stratifin , which are highly expressed in SE-derived cells ( Fig. 6a–d ). IRF6 is a transcription factor, known to be regulated by TFAP2a [28] , which coordinates keratinocyte and breast epithelium proliferation and differentiation [29] , [30] . Stratifin is a member of the 14-3-3 protein family, which functions as an adaptor protein and binds to phosphorylated proteins mediating diverse cellular processes, such as cell cycle control, apoptosis and keratinocyte differentiation [31] . Stratifin promoter DNA hypermethylation and expression downregulation is found in both breast and skin cancers [32] . Mutations in IRF6 or SFN lead to similar phenotypes with limb and craniofacial developmental abnormalities and an impaired skin barrier due to defective keratinocyte differentiation [33] , [34] . Figure 6: RNA expression levels and browser screenshots of selected loci with SE-DMRs. ( a ) Expression values for IRF6 in each cell type as listed on the left; x axis is expression values in log10-transformed RPKM for each cell type. Skin cell-type values are averages (mean) of three biological replicates (error bars are s.e.m. ); luminal epithelial and myoepithelial values are a single biological replicate. ( b ) Browser screenshot of IRF6 locus and surrounding genomic region. MeDIP-seq tracks are shown for the indicated cell types; all track y axes heights are 60 RPKM. Red box, hypomethylated SE-DMR near the IRF6 promoter. ( c ) Expression for Stratifin ( SFN ) as in a . ( d ) Browser screenshot of SFN locus. Tracks as in b . Red box, hypomethylated SE-DMR at SFN promoter. ( e ) Expression values for mir-200c and mir-141 in each cell type as listed to the left; x axis is reads per million (RPM, log scale). Keratinocyte value is the average (mean) of three biological replicates; fibroblast value is the mean of two biological replicates, (error bars are s.e.m. ); melanocyte, luminal epithelial and myoepithelial values are a single biological replicate. ( f ) Browser screenshot of mir-200c/mir-141 locus and surrounding genomic region. Tracks as in b . Red boxes, hypomethylated SE-DMRs including and adjacent to both miRNA loci. Full size image A KLF4 motif containing hypomethylated SE-DMR was noted near the mir-200c/141 locus. These two miRNAs promote epithelial cell fate and mir-200c/141 expression is often lost in breast cancers [35] . Our findings of mir-200c/141 SE-specific expression and DNA hypomethylation ( Fig. 6e,f ) are consistent with previously demonstrated epigenetic regulation of this locus [36] . Thus, SE-DMRs may modulate key genes that regulate proliferation, differentiation and epithelial cell fate maintenance in SE-derived cells. Developmental dynamics of SE regulatory elements To explore the developmental dynamics of DNA methylation at SE-DMRs, we obtained whole-genome bisulfite sequencing (WGBS) data for samples representing early stages in SE development: H1 ESCs and ESCs differentiated to represent an early ectoderm developmental stage [2] . A majority of hypomethylated SE-DMRs were methylated in both early developmental stages, but hypomethylated in keratinocytes and mammary gland epithelia (Methods and Fig. 7a ). The few exceptions are transcription factors that are upstream in the regulatory hierarchy. For example, the DMR near the TFAP2a promoter was demethylated in ESCs, whereas the DMR in KLF4 was methylated in ESCs but demethylated in early SE-differentiated cells. Both genes are most highly expressed in keratinocytes ( Fig. 7b–e ). The remaining hypomethylated SE-DMRs, many of which putatively regulate genes that are TFAP2a, TFAP2c or KLF4 targets in the network analysis, were lowly methylated in differentiated cells. Accordingly, expression of these genes was generally increased in keratinocytes relative to H1 ESCs ( Fig. 7f ). In addition, hypomethylated SE-DMRs were highly methylated in fetal brain tissue, which is predominantly neuroectoderm derived, concordant with their specific assignment to SE-derived cells rather than embryonic ectoderm as a whole ( Supplementary Fig. 10 ). Figure 7: DNA methylation dynamics of SE-DMRs across samples from different developmental stages. ( a ) Heatmap and clustering dendrogram based on average CpG DNA methylation values of hypomethylated SE-DMRs for different developmental samples. Each row represents one of 1,307 DMRs for which there are CpGs with ≥10 × coverage in WGBS data. Methylation values for H1 ESCs, ectoderm differentiated ESCs (‘EC’) and keratinocyte (‘K’) are from WGBS; breast luminal (‘Lu’) and myoepithelial (‘My’) values are the average of single CpG methylCRF predictions in each DMR. MethylCRF predictions are based on MeDIP-seq and MRE-seq data for these samples (Methods). A value of ‘1’ is fully methylated; ‘0’ is completely unmethylated. ( b ) KLF4 gene body SE-DMR average CpG DNA methylation levels across developmental stages. ( c ) KLF4 RNA expression across developmental stages. Values are RPKM over coding exons; error bars for keratinocytes are s.e.m., n =3. Sample abbreviations as in a . ( d ) TFAP2A promoter SE-DMR average CpG DNA methylation levels across developmental stages. ( e ) TFAP2A RNA expression across developmental stages. Values are RPKM over coding exons; error bars for keratinocytes are s.e.m., n =3. Sample abbreviations as in a . ( f ) RNA expression levels in keratinocytes relative to H1 ESCs for selected genes with hypomethylated SE-DMRs in their promoters. These SE-DMRs, as in the majority of hypomethylated SE-DMRs, were methylated in H1 and ectoderm-differentiated ESCs but lowly methylated in differentiated SE cell types. Increased expression relative to an earlier developmental sample suggests these DMRs are transcriptional regulatory regions for their associated genes. Full size image Analysis of an increasingly diverse collection of epigenomes has revealed tissue- and cell type-specific regulatory elements important for cell fate and development [13] , [37] , [38] , [39] , [40] . However, the developmental origins of these epigenomic features have been less explored. Studies using in vitro ESC differentiation systems have uncovered early developmental DNA methylation dynamics that are believed to occur with specification of the embryonic germ layers [1] , [2] . There is a growing realization that this developmental lineage-specific information is maintained in differentiated cells, as DNA methylation and DNase-I-hypersensitive site profiles of cell types and tissues cluster by their embryonic germ layer of origin [6] , [7] . The persistence of a subset of DNA hypomethylated enhancers, which are active in early development but quiescent in adulthood, also suggests a developmental memory is encoded in the epigenome of differentiated cells [6] . Here we present our analysis of the epigenomic features of human skin cell types and their origins. In our experimental design, we used three different skin cell types from the same individual and identified DNA methylation signatures that are consistent for three individuals across each cell type, minimizing variables that confound many other study designs, including genetic background, age and external environmental exposures. Consistent with findings in other cell types, we found many skin cell type-specific DMRs at distal enhancers, enriched for association with cell type-relevant genes, and correlated with expression at hypomethylated promoters. Thus, we demonstrated that, as expected, the cell types within skin tissue possess many regions with cell type-specific epigenomic patterns. Next, we assessed whether the shared environment within skin tissue imparts common epigenomic features on its constituent cell types to create a skin tissue-specific signature. To investigate this question, we developed an approach to identify ‘shared differences’ between epigenomes. This approach prioritized specificity and minimized the influence of variation between biological replicates. Thus, shared epigenomic signatures should be robust to sources of variation and attributable to the common biological factor of the grouped samples; for example, the shared tissue environment of skin cell types. Using this approach on the skin cell-type epigenomes revealed few shared regions compared with epigenomes of other tissues and cell types, suggesting that skin tissue environment had little uniform impact on the epigenomes of its constituent cell types. As tissue environment had minimal effect on skin cell-type epigenomes, we hypothesized that developmental origin may influence differentiated cell epigenomes and confer features specific to their shared origin. We compared the DNA methylomes of SE-derived cells, epidermal keratinocytes and breast luminal and myoepithelial cells, to methylomes of non-SE-derived cells to identify ‘shared differences.’ We found that SE-derived cell types share many DMRs when compared with non-SE-derived cells and that these DMRs possess regulatory potential. This suggests that the common developmental origin of these SE-derived cells impacts their epigenomes, and that this influence is greater than that of tissue environment on keratinocyte methylomes. To gain better insight into the SE-DMR signature, which we defined indirectly through neonatal and adult cell epigenomes, we identified target genes putatively regulated by SE-DMRs and then connected these genes based on known interactions [41] (Methods). The resulting SE network predicted both upstream regulators and co-regulated suites of genes. Transcription factors predicted to bind to SE-DMRs ( Fig. 4c ) were encoded by genes with the highest number of connections in the network ( Supplementary Data 6 and Supplementary Fig. 9 ). The presence of SE-DMRs containing TFAP2 TFBSs near the transcription start site of hemidesmosome genes suggests their co-regulation by TFAP2 family transcription factors. In addition, TFAP2 TFBS-containing SE-DMRs are found near the TSSs of the cell cycle regulators IRF6 and SFN . Given the genetic interaction of these two genes in epidermal development [30] , a TFAP2 motif-binding transcription factor may coordinately co-regulate their expression in SE-derived cells. These examples of predicted regulatory relationships illustrate the significant value afforded by incorporating epigenetically defined regulatory elements into gene networks. A more direct approach to define epigenomic features that arise from a developmental origin would involve isolation and profiling of human embryonic tissues and their derivatives at various time points along a single developmental lineage and comparing their epigenomes and transcriptomes. As this type of experiment is not possible for ethical reasons, we selected cell types arising from a major germ layer derivative, SE, to infer for the first time a DNA methylation signature derived from this inaccessible human embryonic cell population. Our approach builds on previous studies that used induced differentiation of ESCs to elucidate DNA methylation patterns of the three main embryonic germ layers [1] , [2] . Our SE-specific signature findings substantially extend the general concept that epigenomes of differentiated cell types cluster by their embryonic origin [6] , [37] . We demonstrate that a gene network regulating shared biological processes and functional components can be decoded from DNA methylation profiles of cell types specifically chosen for their common embryonic origin. Thus, analysis of differentiated cell types with shared developmental origin may be widely applicable for inference of regulatory epigenomic states derived from other inaccessible precursor human cell populations. Cell type and tissue isolation Fibroblasts, keratinocytes and melanocytes were isolated from neonatal foreskins obtained from circumcision using standard techniques [42] . Briefly, epidermis was mechanically separated from dermis after overnight incubation at 4 °C with dispase solution. The epidermal sheet was incubated with trypsin for 15 min at 37 °C. The disassociated cells were then incubated in selective growth media. Keratinocytes were grown in keratinocyte growth media (Medium 154CF supplemented with 0.07 mM CaCl 2 and Human Keratinocyte Growth Supplement (Life Technologies)). Melanocytes were grown in melanocyte growth media (Medium 254 with Human Melanocyte Growth Supplement (Life Technologies)). Fibroblasts were extracted from the dermis by mincing and digesting with collagenase. The cell suspension was plated in Medium 106 supplemented with Low Serum Growth Supplement (Life Technologies). All skin cell types were harvested after two or three passages by snap freezing in liquid nitrogen. A pure population of keratinocytes was verified by examination of cell morphology and immunofluoresence staining for keratinocyte markers (cytokeratin (acidic), clone AE1, Life Technologies,18-0153) and lack of staining for melanocyte markers (HMB45+Mart-1+Tyrosinase cocktail (Biocare Medical), CM165 or Mel-5 (Covance), Sig-38150). A pure population of melanocytes was verified by examination of cell morphology and immunofluoresence staining for melanocyte markers and lack of staining for keratinocyte markers. A pure population of fibroblasts was verified by examination of cell morphology and positive staining for vimentin (Sigma, V6630) and lack of staining for keratinocyte and melanocyte markers. Breast, blood and fetal brain samples were isolated as previously described [4] . Briefly, for blood cell types, peripheral blood mononuclear cells (PBMCs) were isolated from buffy coat using Histopaque 1077 separation medium (Sigma-Aldrich) according to the manufacturer’s protocol. CD4-naive, CD4-memory and CD8-naive cells were isolated from PBMCs using the following isolation kits: EasySep Human Naive CD4+ T Cell Enrichment Kit, EasySep Human Memory CD4+ T Cell Enrichment Kit and Custom Human Naıve CD8+ T Cell Enrichment Kit (Stemcell Technologies). Pure populations of PBMCs and T-cell subsets were confirmed by staining with the following antibodies (anti-CD3 TRI-COLOR (Invitrogen), anti-CD4 PE (BD Biosciences), anti-CD8 FITC (BD Biosciences), anti-CD4 TRI-COLOR (Invitrogen), anti-CD45RO PE (Invitrogen), anti-CD45RA FITC (BD Biosciences), and anti-CD8 TRI-COLOR (Invitrogen)) and FACS analysis. Briefly, for breast cell types, breast tissue from disease-free premenopausal women was obtained from reduction mammoplasty samples under UCSF CHR protocol 10-01563. Tissue was mechanically and enzymatically dissociated with collagenase and hyaluronidase. Cell suspensions were serially filtered through 150- and 40-μm nylon mesh to obtain epithelial cell enriched clusters (breast cell organoids). To obtain single cell suspensions, organoids were further digested with trypsin and dispase, and filtered with a 40-μm cell strainer followed by incubation for 60–90 min in MEGM medium (Lonza). The resulting cells were stained and sorted by FACS to isolated purified breast myoepithelial and luminal epithelial cells. For positive selection, a PE-Cy7-labelled anti-CD10 antibody (for myoepithelial cells, BD Biosciences, 341092) and a FITC-labelled anti-CD227/MUC1 antibody (for luminal epithelial cells, BD Biosciences, 559774) were used. For negative selection of haematopoietic, endothelial and leukocyte cells, cells were stained with the following antibodies, respectively: anti-CD2, -CD3, CD16, CD64 (BD Biosciences, 555325, 555338, 555405 and 555526); CD31 (Invitrogen, MHCD3115); and CD45, CD140b (BioLegend, 304003 and 323604). Briefly, for fetal brain samples, brain tissue was obtained post-mortem from fetuses whose death was attributed to environmental/placental aetiology, under Partner’s Healthcare/Brigham and Women’s Hospital IRB Protocol 2010P001144. Fetal brain germinal matrix was grossly dissected. Genomic DNA isolation Cells were lysed in extraction buffer (50 mM Tris (pH 8.0), 1 mM EDTA (pH 8.0), 0.5% SDS, and 1 mg ml −1 proteinase K) at 55 °C for 12–16 h. The lysed cells were incubated with 40 μg ml −1 of RNase A for 1 h at 37 °C to remove RNA. DNA was purified by two rounds of phenol/chloroform/isoamyl alcohol extractions and then two rounds of chloroform extractions. DNA was precipitated with 1/10 volume of 3 M sodium acetate (pH 5.2) and 2.5 volumes of ethanol, washed in 70% ethanol and resuspended in TE buffer. Methylation-sensitive restriction enzyme-seq Methylation-sensitive restriction enzyme (MRE)-seq was performed as in Maunakea et al. [43] , with modifications as detailed below. Five parallel restriction enzyme digestions ((HpaII, Bsh1236I, SsiI(AciI) and Hin6I (Fermentas), and HpyCH4IV (NEB)) were performed, each using 1 μg of DNA per digest for each of the skin cell type samples. Five units of enzyme were initially incubated with DNA for 3 h and then an additional five units of enzyme was added to the digestion for a total of 6 h of digestion time. DNA was purified by phenol/chloroform/isoamyl alcohol extraction, followed by chloroform extraction using phase lock gels. Digested DNA from the different reactions was combined and precipitated with 1/10 volume of 3 M sodium acetate (pH 5.2) and 2.5 volumes of ethanol. The purified DNA was size selected and purified (50–300 bp) by gel electrophoresis and Qiagen MinElute extraction. Library construction was performed as per the Illumina Genomic DNA Sample Prep Kit protocol with the following modifications. During the end repair reaction, T4 DNA polymerase and T4 PNK were excluded and 1 μl of 1:5 diluted Klenow DNA polymerase was used. For the adapter ligation reaction, 1 μl of 1:10 diluted PE adapter oligo mix was used. Ten microlitres from the 30 μl of purified adapter ligated DNA was used for the PCR enrichment reaction with PCR PE Primers 1.0 and 2.0. PCR products were size selected and purified (170–420 bp) by gel electrophoresis and Qiagen Qiaquick extraction. DNA libraries were checked for quality by Nanodrop (Thermo Scientific) and Agilent DNA Bioanalyzer (Agilent). Reads were aligned to hg19 using the Burrows-Wheeler Alignment tool (BWA) and pre-processed using methylQA (an unpublished C programme; available at http://methylqa.sourceforge.net/ ). MRE reads were normalized to account for differing enzyme efficiencies and methylation values were determined by counting reads with CpGs at fragment ends [43] . To enable comparison between MRE-seq data from blood, brain and breast samples that used three restriction enzymes and skin cell types that used five restriction enzymes, skin cell-type MRE reads that resulted from the use of additional restriction enzymes (Bsh1236I and HpyCH4IV) were removed. Detailed library construction protocols for MRE-seq, methylated DNA immunoprecipitation-seq (MeDIP-seq), ChIP-seq, RNA-seq and miRNA-seq are publicly available at the NIH Roadmap Epigenomics project website http://www.roadmapepigenomics.org/protocols/type/experimental/ . Methylated DNA immunoprecipitation-seq MeDIP-seq was performed as in Maunakea et al. [43] Five micrograms of genomic DNA was sonicated to a fragment size of ~100–400 bp using a Bioruptor sonicator (Diagenode). End-repair, addition of 3′-A bases and PE adapter ligation with 2 μg of sonicated DNA was performed as per the Illumina Genomic DNA Sample Prep Kit protocol. Adapter-ligated DNA fragments were size selected to 166–366 bp and purified by gel electrophoresis. DNA was heat denatured and then immunoprecipitated with 5-methylcytidine antibody (Eurogentec) (1 μg of antibody per 1 μg of DNA) in 500 μl of immunoprecipitation buffer (10 μM sodium phosphate, pH 7.0, 140 mM sodium chloride and 0.05% Triton X-100) overnight at 4 °C. Antibody/DNA complexes were isolated by addition of 1 μl of rabbit anti-mouse IgG secondary antibody (2.4 mg ml −1 , Jackson Immunoresearch) and 100 μl protein A/G agarose beads (Pierce Biotechnology) for 2 h at 4 °C. Beads were washed six times with immunoprecipitation buffer and then DNA was eluted in TE buffer with 0.25% SDS and 0.25 mg ml −1 of proteinase K for 2 h at 50 °C. DNA was then purified with the Qiagen Qiaquick kit and eluted in 30 μl EB buffer. Ten microlitres of DNA was used for a PCR enrichment reaction with PCR PE Primers 1.0 and 2.0. PCR products were size selected (220–420 bp) and purified by gel electrophoresis. Methylated DNA enrichment was confirmed by PCR on known methylated (SNRPN and MAGEA1 promoters) and unmethylated (a CpG-less sequence on chromosome 15 and glyceraldehyde 3-phosphate dehydrogenase promoter) sequences. DNA libraries were checked for quality by Nanodrop (Thermo Scientific) and Agilent DNA Bioanalyzer (Agilent). Reads were aligned to hg19 using BWA and pre-processed using methlyQA. methylCRF Genome-wide DNA methylation value predictions were made using a conditional random field model that integrates MRE and MeDIP sequencing data for a given sample. The programme was run using default parameters [44] and can be downloaded from http://methylcrf.wustl.edu/ . In Fig. 7 , methylCRF predicted values were averaged for each DMR. Differential DNA-methylated region analysis The M&M statistical model [4] , which integrates MeDIP-seq and MRE-seq data to identify differentially methylated regions between two samples was implemented with a window size of 500 bp and a q -value (false discovery rate (FDR)-corrected P -value) cutoff=1e−5. Scripts used for pairwise comparison are shown in Supplementary Note 2 . Adjacent 500 bp DMRs were merged into a single DMR for further analysis unless otherwise noted. The specific pairwise comparisons performed to generate each DMR set are summarized in Supplementary Fig. 4 . Additional details and discussion of the DMR calling strategy and FDR for M&M analyses are in Supplementary Notes 1 and 3 . Comprehensive lists of identified skin cell-type-specific DMRs are available online ( http://epigenome.wustl.edu/SE ). Whole-genome bisulfite sequencing One to 5 μg of Qubit quantified genomic DNA was used for library construction. Unmethylated Lambda DNA (Promega) was added to genomic DNA for a 0.1% final concentration. DNA was fragmented to ~300 bp using Covaris E series shearing. End-repair, addition of 3′-A bases and adapter ligation was performed as per the Illumina PE Genomic DNA Sample Prep Kit protocol, except that methylated cytosine PE adapters were used. After each of the previous steps, DNA was purified using Ampure XP beads (Agencourt). Bisulfite conversion of purified adapter-ligated DNA was performed using the Epitect bisulfite kit (Qiagen) according to the manufacturer’s instructions. The DNA was amplified by PCR enrichment using Kapa HiFi Hot Start Uracil+Ready (Kapa Biosystems) for five cycles with PCR PE primers 1.0 and 2.0. PCR products were purified with the Qiagen Minelute kit and size selected with PAGE gel purification. DNA libraries were checked for quantity by Qubit (Life Technologies) and quality by Agilent DNA Bioanalyzer (Agilent). Libraries were sequenced using paired-end 100 nt sequencing chemistry on an Illumina HiSeq2000 following the manufacturer’s protocols (Illumina). Raw WGBS sequences were examined for quality, sample swap and reagent contamination using custom in-house scripts. Sequence reads were directionally aligned to the human genome (GRCh37-lite) using Bismark [45] (v. 0.7.6) running Bowtie [45] (v. 0.12.5), allowing up to two mismatches in the 50-bp seed region (using -n 2-l 50 parameters). Methylation status for each aligned CpG was calculated using Bismark Methylation Extractor (v. 0.7.10) at a minimum of 5 × coverage per site in a strand-specific manner (run-time parameters: -p, no_overlap, --comprehensive, --bedGraph, --counts). Overlapping methylation calls from read_1 and read_2 were scored once. All WGBS data was processed using custom scripts to obtain CpG methylation values. CpG methylation values were filtered such that only CpGs with 10 × coverage were subsequently averaged for each DMR in each sample. Lowly methylated regions were called as DMRs for which the average CpG methylation values were ≤0.3. Averaged values were plotted as in Fig. 7 using the R package pheatmaps . Chromatin immunoprecipitation sequencing Standard operating procedures for ChIP-seq library construction are available at http://www.roadmapepigenomics.org/protocols/type/experimental/ . ChIP-seq library construction involves the following protocols in order: (1) cross-linking of frozen cell pellet, (2) DNA sonication using Sonic Dismembrator 550 and (3) SLX-PET protocol for Illumina sample prep. Antibodies used in this study were subjected to rigorous quality assessment to meet Reference Epigenome Mapping Quality Standards ( http://www.roadmapepigenomics.org/protocols ) including western blotting of whole cell extracts, 384 peptide dot blot (Active Motif MODified Histone Peptide Array) and ChIP-seq using control cell pellets (HL60). Antibody vendor, catalogue number and lot are provided along with ChIP-seq library construction details as part of the metadata associated with all ChIP-seq data sets and are available through GEO and the NCBI epigenomics portals (for example, http://www.ncbi.nlm.nih.gov/geo/query/acc.cgi?acc = GSM669589). Final library distributions were calculated using an Agilent Bioanalyzer and quantified by fluorometric quantification (Qubit, Life Technologies). Libraries were sequenced using single-end 76 nt sequencing chemistry on an Illumina GAiix or HiSeq2000 following manufacturer’s protocols (Illumina) as either single or multiplexed libraries using custom index adapters added during library construction. Sequencing reads were aligned to NCBI GRCh37-lite reference using BWA 0.6.2-r126 with default parameters. MethylQA (an unpublished C programme; available at http://methylqa.sourceforge.net/ ) was used to directionally extend aligned reads to the average insert size of DNA fragments (150 bp) and to generate a bigWig file for downstream visualization. Reads with BWA mapping quality scores ≪ 10 were discarded and reads that aligned to the same genomic coordinate were counted only once. Differential ChIP-seq enrichment analysis Mapped read density was generated from aligned sequencing reads using methlyQA. Read density overlapping DMRs and their 5 kb upstream/downstream regions were extracted at 50 bp resolution as reads per kilobase per million mapped reads (RPKM) values. The default parameters were used to apply MACS2 [46] to histone modification ChIP-seq data for the identification of peaks at a 1% FDR. A DMR was defined as enriched for histone signal when at least 60% of the DMR overlapped with histone peaks. Skin cell-type-specific histone peaks were identified using the following two criteria: (1) peaks were identified in at least two of three biological replicates of a skin cell type and (2) peaks were not identified in any of the other two skin cell types or other tissue types (brain, breast and blood). Skin tissue-specific histone peaks were identified using the following three criteria: (1) peaks were identified in at least two of three biological replicates of a skin cell type, (2) peaks were identified in all three skin cell types and (3) peaks were not identified in any other tissue type (brain, breast or blood). Genomic features CpG islands, gene bodies and RefSeq gene annotations (including 5′ and 3′ untranslated regionss, exons and introns) were downloaded from the UCSC Genome Browser. Promoters were defined as the 3.5 kb surrounding the TSS (−3 kb/+500 bp) of all RefSeq genes. Intergenic regions were defined as all regions outside RefSeq gene bodies and promoters. GO enrichment analysis GO analyses for biological processes were performed using the GREAT package [14] . Gene regulatory domains were defined by default as the regions spanning 5 kb upstream and 1 kb downstream of the TSS (regardless of other nearby genes). Gene regulatory domains were extended in both directions to the nearest gene’s basal domain, but no more than a maximum extension in one direction. Only categories that were below an FDR of 0.05 were reported. TFBS identification enrichment Genome sequences were obtained for hypomethylated SE-DMRs from the hg19 human genome assembly. Motif finding analysis was performed using the FIMO tool from the MEME suite and default vertebrate databases [47] , [48] , with a q -value (FDR-corrected P -value) cutoff of 0.04 Motif enrichment was calculated as the number of motif instances found in the test data compared with the number found genome wide (for hg19), normalized for length. where n DMRs =number of a given motif found in the hypomethylated SE-DMRs and N hg19 =number of a given motif found in hg19; 820,000=number of base pairs in hypomethylated SE-DMRs and 3,200,000,000=number of base pairs in the human genome. Regulatory network construction Regulatory networks were constructed in the following steps. First, genes (nodes) were identified as putative targets of regulatory (hypomethylated) SE-DMRs either by their association with DMRs that fell in the promoter region of RefSeq genes (−3 kb/+500 bp TSS) or by association as distal intergenic regulatory elements. Intergenic DMRs were associated with genes whose TSS fell in a window of ±35 kb (this window size is chosen based on literature assessing the average distance of enhancer–promoter associations [38] ). The collection of these promoter- and distal enhancer-associated gene lists were then filtered for a gene expression level ≥1 RPKM in any of the SE-derived cell types; for the SE network this resulted in 374 genes. To obtain interactions between genes in this list, the gene list was used as nodes in the UCSC Interaction Browser [41] . The Interaction Browser queries known databases for connections (links) between a given set of genes (nodes). Four pathway collections (GEA_CLR TF-targets network, UCSC_Superpathway, UCSC_Superpathway_collapsed and CHEA transcription factors) were used to query for interactions between the given genes. For the SE-DMR network, KLF4 was added to the gene list because its motif was enriched in hypomethylated SE-DMRs ( Fig. 4c ) and because it is known to be important for keratinocyte differentiation [49] . Klf4 does have two hypomethylated SE-DMRs in its second exon, suggesting it is regulated, but the exonic location of the Klf4 DMRs excluded it from the stringent method for identifying putatively regulated genes above. Similarly, TFAP2C was added to the gene list, because it is known to be important in keratinocyte differentiation [16] and its motif (shared with TFAP2A) was enriched in our motif analysis ( Fig. 4c ). For the network overview presented in Fig. 5a , the transcription factor p63 was added at the top of the network, as it integrates both network branches, is a known regulator of the ZNF750–KLF4 transcriptional cascade [50] and interacts genetically with TFAP2a/c [51] , [52] ; however, p63 and its edges are not included in the data ( Supplementary Data 6 ) or network structural analysis ( Supplementary Table 7 and Supplementary Fig. 9 ). We applied the same method for generating links between a set of 374 random genes to obtain an expected distribution of links given the number of genes in the test network. This resulted in a distribution as described in Supplementary Table 7 , with a mean of 958 and variance of 136.5. By a t -test, the number of links in the SE network is statistically significant ( P -value=1.245e−4). To assess the scale-free properties of the SE network, we calculated the number of edges assigned to each node and plotted this distribution in Supplementary Fig. 9 . Accession codes: Accession codes for keratinocyte skin01 MeDIP-seq, MRE-seq, mRNA-seq, miRNA-seq, H3K4me3 ChIP-seq, H3K4me1 ChIP-seq and input ChIP-seq data sets have been deposited in the Gene Expression Omnibus (GEO) database under the accession codes GSM707022 , GSM707018 , GSM751278 , GSM817253 , GSM66958 , GSM669591 and GSM817242 , respectively. Accession codes for keratinocyte skin02 MeDIP-seq, MRE-seq, mRNA-seq, miRNA-seq, H3K4me3 ChIP-seq, H3K4me1 ChIP-seq and input ChIP-seq data sets have been deposited in the GEO database under the accession codes GSM941726 , GSM941723 , GSM941745 , GSM1127113 , GSM941735 , GSM941736 and GSM941742 , respectively. Accession codes for keratinocyte skin03 MeDIP-seq, MRE-seq, mRNA-seq, miRNA-seq, WGBS, H3K4me3 ChIP-seq, H3K4me1 ChIP-seq, H3K27ac ChIP-seq and input ChIP-seq data sets have been deposited in the GEO database under the accession codes GSM958180 , GSM958169 , GSM958177 , GSM1127111 , GSM1127056 / GSM1127058 , GSM958155 , GSM958161 , GSM958156 and GSM958167 , respectively. Accession codes for fibroblast skin01 MeDIP-seq, MRE-seq, mRNA-seq, miRNA-seq, H3K4me3 ChIP-seq, H3K4me1 ChIP-seq and input ChIP-seq data sets have been deposited in the GEO database under the accession codes GSM707021 , GSM707017 , GSM751277 , GSM817252 , GSM817235 , GSM817234 and GSM817246 , respectively. Accession codes for fibroblast skin02 MeDIP-seq, MRE-seq, mRNA-seq, H3K4me3 ChIP-seq, H3K4me1 ChIP-seq and input ChIP-seq data sets have been deposited in the GEO database under the accession codes GSM941725 , GSM941722 , GSM941744 , GSM941718 , GSM941717 and GSM817247 , respectively. Accession codes for fibroblast skin03 MeDIP-seq, MRE-seq, mRNA-seq, miRNA-seq, H3K4me3 ChIP-seq, H3K4me1 ChIP-seq, H3K27ac ChIP-seq and input ChIP-seq data sets have been deposited in the GEO database under the accession codes GSM958182 , GSM958171 , GSM958178 , GSM1127116 , GSM958158 , GSM958164 , GSM958163 and GSM958168 , respectively. Accession codes for melanocyte skin01 MeDIP-seq, MRE-seq, mRNA-seq, miRNA-seq, H3K4me3 ChIP-seq, H3K4me1 ChIP-seq and input ChIP-seq data sets have been deposited in the GEO database under the accession codes GSM707020 , GSM707016 , GSM751276 , GSM817251 , GSM941719 , GSM941728 and GSM941740 , respectively. Accession codes for melanocyte skin02 MeDIP-seq, MRE-seq, mRNA-seq, H3K4me3 ChIP-seq, H3K4me1 ChIP-seq and input ChIP-seq data sets have been deposited in the GEO database under the accession codes GSM941727 , GSM941724 , GSM941743 , GSM941731 , GSM941730 and GSM941741 , respectively. Accession codes for melanocyte skin03 MeDIP-seq, MRE-seq, mRNA-seq, H3K4me3 ChIP-seq, H3K4me1 ChIP-seq, H3K27ac ChIP-seq and input ChIP-seq data sets have been deposited in the GEO database under the accession codes GSM958181 , GSM958170 , GSM958174 , GSM958151 , GSM958152 , GSM958157 and GSM958166 , respectively. Accession codes for breast luminal epithelia RM071 MeDIP-seq and MRE-seq data sets have been deposited in the GEO database under the accession codes GSM1517154 and GSM613826 , respectively. Accession codes for breast luminal epithelia RM080 mRNA-seq, H3k4me1 ChIP-seq and input ChIP-seq data sets have been deposited in the GEO database under the accession codes GSM669620 , GSM669595 and GSM959124 , respectively. Accession codes for breast myoepithelia RM071 MeDIP-seq and MRE-seq data sets have been deposited in the GEO database under the accession codes GSM1517153 and GSM613908 , respectively. Accession codes for breast myoepithelia RM080 H3K4me3 ChIP-seq, H3k4me1 ChIP-seq and input ChIP-seq data sets have been deposited in the GEO database under the accession codes GSM693277 , GSM613885 and GSM613897 , respectively. Accession codes for the Fetal Brain Germinal Matrix HuFGM02 WGBS data set have been deposited in the GEO database under the accession code GSM941747 . Accession codes for PBMC TC015 H3K4me3 ChIP-seq, H3k4me1 ChIP-seq and input ChIP-seq data sets have been deposited in the GEO database under the accession codes GSM613811 , GSM613814 and GSM613816 , respectively. Accession codes for CD8 Naive TC001 H3K4me3 ChIP-seq, H3k4me1 ChIP-seq and input ChIP-seq data sets have been deposited in the GEO database under the accession codes GSM1127126 , GSM1127143 and GSM1127151 , respectively. How to cite this article : Lowdon, R. F. et al. Regulatory network decoded from epigenomes of surface ectoderm-derived cell types. Nat. Commun. 5:5442 doi: 10.1038/ncomms6442 (2014).